Broadband terahertz generation from metamaterials The terahertz spectral regime, ranging from about 0.1–15 THz, is one of the least explored yet most technologically transformative spectral regions. One current challenge is to develop efficient and compact terahertz emitters/detectors with a broadband and gapless spectrum that can be tailored for various pump photon energies. Here we demonstrate efficient single-cycle broadband THz generation, ranging from about 0.1–4 THz, from a thin layer of split-ring resonators with few tens of nanometers thickness by pumping at the telecommunications wavelength of 1.5 μm (200 THz). The terahertz emission arises from exciting the magnetic-dipole resonance of the split-ring resonators and quickly decreases under off-resonance pumping. This, together with pump polarization dependence and power scaling of the terahertz emission, identifies the role of optically induced nonlinear currents in split-ring resonators. We also reveal a giant sheet nonlinear susceptibility ~10 −16 m 2 V −1 that far exceeds thin films and bulk non-centrosymmetric materials. The challenge to develop and apply terahertz (THz) light sources merges different disciplines of fundamental science and technology, ranging from ultrafast nonlinear optics, condensed matter and material physics to optoelectronics and microwave photonics. The emerging THz technologies, such as quantum-cascade lasers [1] , [2] , [3] , and ultrafast photoconductive switches [4] , have enabled various THz spectroscopy/imaging/sensing developments and have offered perspectives, among others, for pushing the GHz switching speed limit of today’s logic/memory/wireless communication devices into the THz regime [4] , [5] . The broadband THz spectroscopy approach also potentially opens exciting opportunities to study fundamental correlation physics in advanced materials ranging from nanostructures to strongly correlated electron materials [6] , [7] , [8] . In regard to broadband THz sources, a major recent progress [9] is based on nonlinear optical rectification in inorganic crystals, such as ZnTe/GaP/GaAs/GaSe/DAST/LiNbO 3 , pumped by femtosecond laser pulses combined with field-resolved detection via electro-optic sampling using similar crystals. However, issues in these crystals are strongly absorbing longitudinal optical phonon bands that lead to a gap in the THz spectrum in the Reststrahlen region; subtle quasi-phase-matching conditions that require locking phase velocity of the THz emission to group velocity of the optical pump, which restricts the accessible pump photon energies to a fixed and narrow range in order to increase the coherent length. Recently, there have been efforts on thin THz emitter/detector crystals of 10–30 μm thickness [9] , [10] to increase the THz emission bandwidth by leveraging above-mentioned restrictions and to enable integration with current micro-/optoelectronics technology. However, the relatively small nonlinear susceptibilities of inorganic emitters limit the THz emission intensity. Meanwhile, nonlinear metamaterials have been actively pursued [11] , [12] , [13] , [14] , [15] , [16] , [17] , [18] , [19] , and the recent development of metamaterials composed of split-ring resonators (SRRs) has enabled researchers to tailor resonant optical nonlinearities from the THz to the infrared and visible regions [20] , [21] . In this regard, investigating metamaterials with few tens of nanometres thickness exhibiting artificial optical magnetism—that is, sustaining circulating ring currents at optical frequencies—can meet the urgent demand for new nonlinear materials for optical rectification free from both quasi-phase-matching limitation and spurious THz phonon absorption. This is mainly due to the coexistence of resonant nonlinearity [22] , [23] , [24] from magnetic dipoles and local electric field enhancement in the narrow gaps of the SRRs, which together allows efficient and broadband THz radiation from emitters of significantly reduced thickness. In addition, tailoring the magnetic resonances of the metamaterial emitters allows for matching to essentially any desired pump photon energy. For example, this allows integration of THz optoelectronics with high-speed telecommunications as the 1.3–1.5 μm range is not ideal for the above inorganic crystals. Some other nonlinear media have also been explored, although they mostly suffer from either poor stability or limited bandwidth, for example, bulky ambient air-plasma generation normally with large shot-by-shot fluctuations [25] , [26] , and electrically-biased photoconductive antennas that not only require extra voltage driving sources but also have limited bandwidth [27] ; some substrate materials such as GaAs still have strong TO and LO phonon resonances at 8.1 and 8.8 THz, which limits the THz radiation in this range [28] . The same narrow THz emission bandwidth has also been seen from femtosecond-laser-accelerated photoelectrons in nano-plasmonic structures [29] , [30] . In this Article, we demonstrate efficient THz emission up to 4 THz from optical rectification in a single-SRR layer of 40 nm in thickness, based on resonant photoexcitation of the magnetic-dipole resonance centred around 1,500 nm wavelength using 140 fs laser pulse. The strong THz emission amplitude from the metamaterial is on the same order as optimal ZnTe crystals that are thousands of times thicker, revealing a gigantic resonant second-order sheet nonlinear susceptibility of SRRs ~10 −16 m 2 V −1 , which is three orders of magnitude higher than the typical surface and sheet values of bulk crystals and thin films [31] , [32] , [33] . 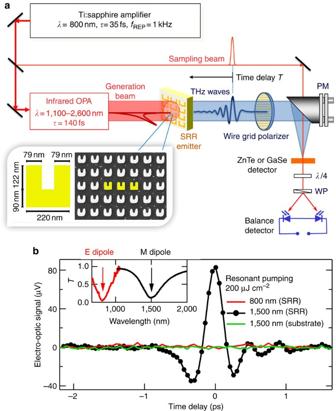Figure 1: Experimental setup and measured THz signals. (a) Schematics of THz generation and detection. The magnified frame at the bottom left shows an electron micrograph of the SRR array along with yellow SRR overlays being the design geometry of the SRRs. PM: parabolic mirror, WP: Wollaston prism. (b) Measured THz time-domain signals by pumping the SRR electric-dipole resonance (red line) at 800 nm, magnetic-dipole resonance (black dots) at 1,500 nm and pure substrate (green line) at 1,500 nm, respectively. The inset exhibits the linear optical transmission showing electric (red curve) and magnetic (black curve) dipole resonances of the SRRs. They are measured with the polarization of the incident light either perpendicular (electric) or parallel (magnetic) to the gap of SRRs. Experimental setup and sample characteristics Figure 1a schematically illustrates the experiment and shows key elements. A Ti:sapphire amplifier is used to drive the whole setup with center wavelength 800 nm, pulse duration 35 fs and repetition rate 1 kHz. The main portion of the output from the amplifier is used to pump an optical parametric amplifier (OPA) to produce tunable near-infrared (NIR) radiation from 1,100 to 2,600 nm of about 140 fs pulse duration. The NIR radiation from the OPA is used as a generation beam to pump the metamaterial emitter made of a single layer of 40 nm thin SRRs. The generated THz pulses are focused onto a ZnTe or GaSe crystal by a parabolic mirror for electro-optic sampling by a small portion of the amplifier output. A wire grid polarizer is used to measure the polarization of the generated THz pulses. An electron micrograph of the metamaterial SRR array is shown in the magnified frame at the bottom left of Fig. 1a . The sample has been fabricated using electron-beam lithography and high-vacuum evaporation of gold, followed by a lift-off procedure. The sample is composed of a single layer of 40 nm thin gold SRRs with a square lattice constant of 382 nm on a 1 mm thick suprasil substrate, coated with a 5 nm thin ITO layer that serves to prevent distortion due to local charge accumulation during the e-beam lithography. The big yellow SRR on the left illustrates the geometrical parameters used for the numerical calculations. Three small yellow SRRs are overlaid in the middle of SRR array micrograph in order to compare the designed SRR geometry with the actual SRR dimension. Figure 1: Experimental setup and measured THz signals. ( a ) Schematics of THz generation and detection. The magnified frame at the bottom left shows an electron micrograph of the SRR array along with yellow SRR overlays being the design geometry of the SRRs. PM: parabolic mirror, WP: Wollaston prism. ( b ) Measured THz time-domain signals by pumping the SRR electric-dipole resonance (red line) at 800 nm, magnetic-dipole resonance (black dots) at 1,500 nm and pure substrate (green line) at 1,500 nm, respectively. The inset exhibits the linear optical transmission showing electric (red curve) and magnetic (black curve) dipole resonances of the SRRs. They are measured with the polarization of the incident light either perpendicular (electric) or parallel (magnetic) to the gap of SRRs. Full size image THz emission from electric and magnetic-dipole resonances Typical time-domain THz traces, E THz , during the 4-ps interval and for a pump fluence of 200 μJ cm −2 , are shown in Fig. 1b for two pump wavelengths: this clearly demonstrates THz generation exclusively from pumping at the SRR magnetic-dipole resonance (inset, black arrow) with 1,500 nm (black dots), while there is negligible THz signal from pumping at the electric-dipole resonance (inset, red arrow) with 800 nm (red line) and pumping of the bare substrate with 1,500 nm (green line). Note that the two resonances are excited with the linear polarization of the incident pump light either perpendicular (electric) or parallel (magnetic) to the gap of SRRs. In addition, we characterize the polarization state of the emitted THz pulses to be perpendicular to the gap of the SRRs, consistent with the second-order nonlinearity. Pump wavelength dependence of THz generation To further investigate the nature of the THz emission, the false-colour plot and the time-domain THz traces in Fig. 2 show the detailed excitation-wavelength dependence. Resonant photoexcitation of the magnetic-dipole resonance ~1,540 nm leads to significant enhancement of the THz emission, as shown in Fig. 2a . The corresponding time-domain trace for the on-resonance pumping is plotted in Fig. 2c . The conversion efficiency quickly decreases under off-resonance pumping, which is shown by the reduction of the THz emission for excitation both below and above the magnetic-dipole resonance, at 2,180 nm ( Fig. 2b ) and 1,376 nm wavelengths ( Fig. 2d ), respectively. The peak-to-peak amplitudes of THz emission Δ E THz (red diamonds) closely follow the absorption around the magnetic-dipole resonance, as seen by comparison with the 1− T curve (blue, left side panel, Fig. 2a ), where T is the linear optical transmission of the sample. All of these observations corroborate the resonant THz generation from nonlinear currents induced by the electrically coupled fundamental magnetic SRR resonance. 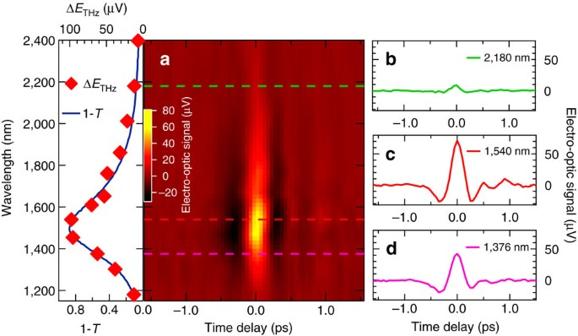Figure 2: Pump wavelength dependence of THz generation from the SRR metamaterial. (a) A two-dimensional false-colour plot of the THz temporal traces for sweeping the pump wavelength across the magnetic-dipole resonance. The left-hand-side panel summarizes peak-to-peak amplitudes of THz emission (red diamonds) as a function of pump wavelength, together with the 1−Tcurve (blue solid line).Tis the measured transmission around the SRR’s magnetic-dipole resonance. The three coloured curves (green, red, magenta) indicate the cut positions of three time-domain traces shown in (b–d) corresponding to 2,180 nm, 1,540 nm and 1,376 nm, respectively. If the pump wavelength is detuned from the resonance, the signal amplitude quickly decreases and the line shape matches very well with the 1−Tcurve. Figure 2: Pump wavelength dependence of THz generation from the SRR metamaterial. ( a ) A two-dimensional false-colour plot of the THz temporal traces for sweeping the pump wavelength across the magnetic-dipole resonance. The left-hand-side panel summarizes peak-to-peak amplitudes of THz emission (red diamonds) as a function of pump wavelength, together with the 1− T curve (blue solid line). T is the measured transmission around the SRR’s magnetic-dipole resonance. The three coloured curves (green, red, magenta) indicate the cut positions of three time-domain traces shown in ( b – d ) corresponding to 2,180 nm, 1,540 nm and 1,376 nm, respectively. If the pump wavelength is detuned from the resonance, the signal amplitude quickly decreases and the line shape matches very well with the 1− T curve. 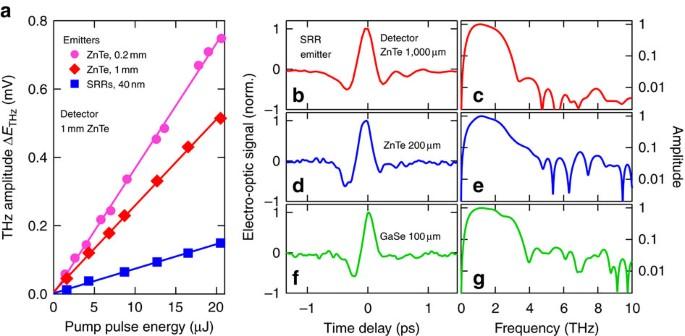Figure 3: Comparison of emitters and measured spectral bandwidths. (a) The peak-to-peak amplitude of THz signal versus pump power measured with three different THz emitters: 0.2 mm ZnTe (magenta dots), 1 mm ZnTe (red diamonds) and SRR (blue squares) and the same detector of 1 mm ZnTe. The straight lines are from linear fitting. (b–g) The normalized time-domain THz pulses and corresponding spectral amplitudes generated from the SRR emitter and three different detectors. (b,c) 1 mm ZnTe detector (red); (d,e): 0.2 mm ZnTe (blue); (f,g): 0.1 mm GaSe (green). Full size image Comparison of SRRs with other emitters Figure 3a compares the peak-to-peak amplitude of THz electric field Δ E THz versus pump power for the single layer 40 nm SRR emitter (blue squares) with two ZnTe emitters with thicknesses of 1 mm (red diamonds) and 0.2 mm (magenta dots), respectively. The THz signals for the three emitters are measured at the same pump fluence and using the same ZnTe detector crystal of 1 mm in thickness. For the ZnTe emitters pumped at 1,500 nm, coherence length L c for the THz emission is ~0.2 mm (ref. 28 ). Increasing the crystal thickness beyond this value actually decreases the emission intensity, as seen for the 1 mm ZnTe case. This effect is expected from the quasi-phase-matching in the ZnTe emitter crystal: after propagating L c , the superposition of the emitted THz pulses from different sheets will have destructive interference in the ZnTe. Most intriguingly, Fig. 3a reveals a remarkably efficient THz generation from the single layer of SRRs with emission intensity on the same order as the optimal ZnTe emitters of 5,000 times thicker: the SRRs generate THz radiation approximately one-fifth of the maximum from the 0.2 mm ZnTe. The emitted THz electric field scales linearly with the pump power, which corroborates the optical rectification process. Our phase-resolved THz measurements from the SRR and ZnTe emitters allow us to unambiguously determine the second-order nonlinear susceptibility of a single-SRR layer to be 0.8 × 10 −16 m 2 V −1 (see Supplementary Note 1 ), which has not been possible from previous nonlinear measurements such as second-harmonic generation (SHG) [22] , [23] . Figure 3: Comparison of emitters and measured spectral bandwidths. ( a ) The peak-to-peak amplitude of THz signal versus pump power measured with three different THz emitters: 0.2 mm ZnTe (magenta dots), 1 mm ZnTe (red diamonds) and SRR (blue squares) and the same detector of 1 mm ZnTe. The straight lines are from linear fitting. ( b – g ) The normalized time-domain THz pulses and corresponding spectral amplitudes generated from the SRR emitter and three different detectors. ( b , c ) 1 mm ZnTe detector (red); ( d , e ): 0.2 mm ZnTe (blue); ( f , g ): 0.1 mm GaSe (green). Full size image Figure 3b–g plots normalized temporal profiles of THz electric fields and corresponding spectral amplitudes from the single layer SRR emitter. The THz detector crystals are 1 mm ZnTe (red, Fig. 3b,c ), 0.2 mm ZnTe (blue, Fig. 3d,e ) and 0.1 mm GaSe detector (green, Fig. 3f,g ). This demonstrates the THz bandwidth of the SRR emitter up to 4 THz that is limited mostly by the excitation pulse of duration ~140 fs (spectral width ~13 meV or 3.2 THz) and by the Reststrahlen region of the inorganic nonlinear detector crystals (centred ~5–6 THz). Our approach can potentially even generate much higher THz bandwidth by shortening the pump pulses because the single-layer SRR emitter does not suffer from the intrinsic limitation of the Reststrahlen region in almost all inorganic THz emitters/sensors. 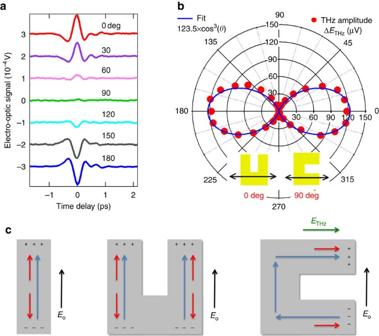Figure 4: Polarization dependence of THz generation from SRRs. (a) The THz signals measured at several angles between the polarization of 1,500 nm pump beam and the gaps of SRRs. The traces are offset for clarity. (b) The polar graph of the peak-to-peak amplitudes of THz signals as a function of the SRR emitter rotation angle. The inset defines the angles between the polarization of the 1,500 nm pump beam (black arrows) and the SRRs. (c) Distributions of the linear current (blue), nonlinear polarization (red) for a linear cut-wire (left) as well as the electric resonance (middle) and electrically excited magnetic resonance (right) of the SRR. The + and − indicate charge accumulation. Only one of them, the magnetic resonance of the SRR (right), exhibits an appreciable THz (green) via optical rectification due to the broken symmetry. Polarization dependence of THz generation Figure 4a shows the control of the amplitude and phase of THz emission by varying relative polarization by rotating the SRR emitter. As shown in the inset of Fig. 4b , we define the polarization angle to be 0 degree when the polarization of the pump beam is parallel to the gap of the SRR and 90 degrees for the orthogonal polarization. Figure 4a plots 7 traces by varying the SRR emitter from 0 to 180 degree under 1,500 nm pumping (traces are offset for clarity). It clearly shows that the THz emission amplitude oscillates starting from a maximum at 0 degree, crosses zero at 90 degrees and returns back to a maximum at 180 degrees with a π phase shift from the origin. The complete polarization dependence of the emission amplitude is shown as a polar graph in Fig. 4b where the peak-to-peak amplitude of THz signal is plotted as a function of the rotation angle. The amplitude is best fitted with a cos 3 ( θ ) function, where a cos 2 ( θ ) dependence is from the polarization between the pump beam and the gap of the SRR, and the other cos( θ ) originates from the detection ZnTe crystal. In short, the detector is aligned such that it measures vertically (horizontally) polarized THz pulses at maximum (minimum) efficiency and the efficiency follows a cos( θ ) function [34] . Figure 4: Polarization dependence of THz generation from SRRs. ( a ) The THz signals measured at several angles between the polarization of 1,500 nm pump beam and the gaps of SRRs. The traces are offset for clarity. ( b ) The polar graph of the peak-to-peak amplitudes of THz signals as a function of the SRR emitter rotation angle. The inset defines the angles between the polarization of the 1,500 nm pump beam (black arrows) and the SRRs. ( c ) Distributions of the linear current (blue), nonlinear polarization (red) for a linear cut-wire (left) as well as the electric resonance (middle) and electrically excited magnetic resonance (right) of the SRR. The + and − indicate charge accumulation. Only one of them, the magnetic resonance of the SRR (right), exhibits an appreciable THz (green) via optical rectification due to the broken symmetry. Full size image Optical rectification, responsible for the observed THz emission, is induced by the broken symmetry in the second-order nonlinear current distribution, which arises exclusively from the photoexcited magnetic-dipole resonance of the SRR. The second-order nonlinearities for the metallic response can be described by a hydrodynamic model [24] known as Maxwell-Vlassov theory. It treats the main nonlinear second-order contributions originating from the and terms, which do not contribute in the bulk but do contribute on surfaces (see Supplementary Note 2 ). Both terms can induce the nonlinear current either parallel or antiparallel to the linear current induced by the external excitation in regions of increasing or decreasing surface charge, respectively, as illustrated in Fig. 4c . In the case of a simple straight nanorod (left panel), the radiations caused by the nonlinear current contribution (red) in the two regions of surface charge accumulation (that is, both ends of the nanorod) are out of phase and thereby interfere destructively. Therefore, no emission is observable in the far field. Similarly, the symmetry of the current distribution at the electric-dipole resonance of the SRR (middle panel) cannot induce radiation either. If, however, one bends the nanorod into a U-shaped SRR and excites the magnetic resonant mode (right panel) that has a continuous current (without nodes) around the SRR ring, the nonlinear current in both arms are now parallel and their radiated fields interfere constructively. This leads to the observed THz emission in the far field perpendicular to the SRR gap (green line). It should be noted that, although this mechanism also works for the SHG reported previously [22] , [23] , the current phase-resolved THz results allow us to quantitatively reveal the nonlinear susceptibility of the SRRs previously inaccessible and phase reversal of THz emission. Next, we make a brief comparison between our approach and the previous THz generation work in nano-plasmonic structures, for example, as shown in ref. 29 (see Supplementary Note 3 for details). This clearly shows not only the distinctly different nonlinear mechanisms involved in the THz generation processes but also the new findings in our work over the previous work. First, our work demonstrates THz generation, ranging from 0.1 to 4 THz, free from quasi-phase-matching and phonon limitations. This bandwidth is mostly limited by the excitation pulse of duration ~140 fs (spectral width ~3.2 THz). In contrast, ref. 29 , with shorter pulse duration (broader spectral width), demonstrates bandwidth less than 1.5 THz. This shows the scheme there still suffers from those conventional limitations unlike the demonstration in our work. Second, the distinctly different power dependence of the THz emission between our SRRs and the silver nanoparticle work at similar excitation intensity clearly indicates the different optical nonlinear mechanism used. Our work also reveals more aspects of nonlinear optical phenomena ranging from distinct electric versus magnetic-dipole excitation dependence and polarization control to resonant enhancement and pump photon energy selectivity, all of which are rarely addressed in any other platform. Last, our SRR scheme and THz results allow a thorough understanding regarding the THz physics of nonlinear metamaterials. Our results identify the nonlinear mechanism that arises from exciting the magnetic-dipole resonance of SRRs and determine the second-order nonlinear susceptibility of the SRRs. In summary, we show that a single-nanometre scale layer of SRRs merges nonlinear metamaterials and THz science/technology, representing a new platform for exploring artificial-magnetism-induced nonlinear THz generation. This leads to broadband THz emission from deep-subwavelength-scale meta-atoms. Optical measurement In our experiment, a Ti:sapphire amplifier is used with center wavelength 800 nm, pulse duration 35 fs at 1 kHz repetition rate. The main portion of the output from the amplifier is used to pump the OPA to produce tunable NIR radiation from 1,100 to 2,600 nm with ~140 fs pulse duration, which serves as a generation beam to pump the SRR/ZnTe emitter. The FWHM of the NIR beam is ~4 mm. Therefore, 1 μJ pulse energy corresponds to the fluence of 8 μJ cm −2 and an intensity of 5.7 × 10 7 W cm −2 . The generated THz pulses are then focused onto the ZnTe or GaSe detector by a parabolic mirror. Residual scattered NIR radiation from the pump pulse is removed from the THz signal by a Teflon filter before the detector. The other small portion of the output from the amplifier is used as a sampling beam to detect the THz pulses via the electro-optic sampling of the detector crystals. The THz section of the setup is purged with dry N 2 gas. Note the wire grid polarizer shown in Fig. 1a indicates the position where the polarization of generated THz pulses is measured. It is used only for the determination of the polarization and not presented for all the other experiments discussed in the article. For polarization dependence measurements, the SRR emitter is rotated while the NIR pump beam remains fixed, so that the polarization of generated THz pulses is rotated together with SRR emitter accordingly. In addition, the detection ZnTe crystal is also polarized, which explains the cos 3 ( θ ) fitting used in Fig. 4 . How to cite this article: Luo, L. et al. Broadband terahertz generation from metamaterials. Nat. Commun. 5:3055 doi: 10.1038/ncomms4055 (2014).